Skeletal muscle stem cells adopt a dormant cell state post mortem and retain regenerative capacity The accessibility to stem cells from healthy or diseased individuals, and the maintenance of their potency are challenging issues for stem cell biology. Here we report the isolation of viable and functional skeletal myogenic cells from humans up to 17 days, and mice up to 14 days post mortem, much longer beyond previous reports. Muscle stem cells are enriched in post mortem tissue, suggesting a selective survival advantage compared with other cell types. Transplantation of mouse muscle and haematopoietic stem cells regenerates tissues robustly. Cellular quiescence contributes to this cell viability where cells adopt a reversible dormant state characterized by reduced metabolic activity, a prolonged lag phase before the first cell division, elevated levels of reactive oxygen species and a transcriptional status less primed for commitment. Finally, severe hypoxia, or anoxia is critical for maintaining stem cell viability and regenerative capacity. Thus, these cells provide a useful resource for studying stem cell biology. Because of the limited availability of stem cells for experimental manipulations or regenerative medicine, there is a heightened interest in improving the viability of tissue-specific stem cells that can be obtained from a variety of healthy and diseased individuals. However, these potent cells are often rare and only available in small quantities when isolated from patients after tissue biopsy. Furthermore, stem cells are often difficult to purify from other cell types in many cases due to the lack of specific markers. Hence, the isolation of normally occurring populations of stem cells from adult tissues is currently technically difficult and costly. Although some of these obstacles might be overcome, other limitations include shortages in the number of donors, as well as difficulties in finding matching donors, especially for minority groups. Therefore, defining conditions for enriching stem cells from biological material comprising other cell types is critical to facilitate their use for research or use in the clinic. Stem cells from post mortem tissues are currently used for experimentation, yet stem cell viability and regenerative capacity are thought to decline significantly in cadavers, consequently these studies have been limited to about 2 days after death [1] , [2] , [3] , [4] , [5] , [6] , [7] . Here we describe culture conditions that permit the survival and full engraftment potential of muscle and haematopoietic stem cells (HSCs) for remarkably longer periods post mortem than previously described, providing a source of stem cells for use in studying stem cell biology. Viability of human and mouse muscle stem cells post mortem Histological examination of skeletal muscle biopsies from human cadavers at 6–17 days post mortem showed severe autolytic alterations with oedema compared with normal tissue (57–95 years old (y.o. 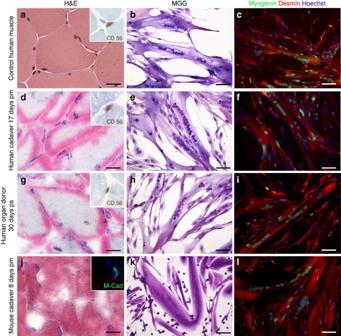Figure 1: Skeletal muscle stem cells survive for extended periods post mortem. Tissue and cells from freshly sampled human biopsy (a–c). (a) Histology. Insets: immunostaining with satellite cell marker (CD56, brown). (b) Myotubesin vitroafter 14 days culture from muscle biopsy (from same patient) expressing myogenin and desmin (c). Human deltoid muscle collected 17 days post mortem (d–f), (d) histology— inset is a CD56+ satellite cell, (e) myotube formation expressing myogenic markers (f). Muscle biopsy stored for 25 days post sampling (ps) from patient (g–i), (g) histology with a CD56+ satellite cell (inset), (h) myotube formation expressing myogenic markers (i). Mouse skeletal TA muscle 8 days post mortem (j–l) (n=10 mice per time point). (j) Histology—inset satellite cell expressing M-Cadherin, (k) myotube formation, expressing myogenin and desmin (l). Note necrosis of haematoxylin and eosin (H&E)-stained myofibres (d–j). Histology figures are H&E stainings. Myotubes are stained with May Grünwald Giemsa (MGG) and immunostained with anti-myogenin (green), anti-desmin (red), and nuclei are counterstained with Hoechst (blue). Bar: 10 μm. ); n =16; Table 1 ). However, examination with markers showed the presence of muscle stem (satellite) cells (CD56 + /N-CAM + ; Fig. 1a,d and insets) [8] . Strikingly, as observed with freshly isolated human muscle stem cells ( Fig. 1b ), in all cases (including 17 days post mortem), culture of dissociated muscle biopsies yielded adherent cells after a maximum of 4 days that differentiated and fused spontaneously ( Fig. 1e ). Immunostaining confirmed that over 90% of the cells expressed Myogenin, a transcription factor specific for muscle differentiation [9] , and the myogenic marker Desmin ( Fig. 1c,f ). We were not able to obtain human cadavers after 17 days post mortem for experimentation. These observations were confirmed with organ donor-derived muscle biopsies that were stored for several days at 4 °C ( Fig. 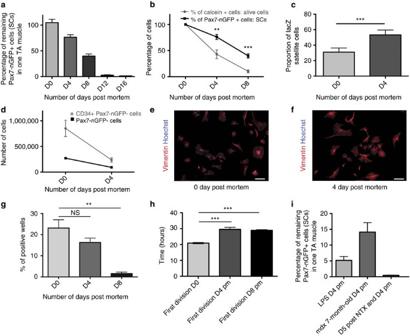Figure 2: Characterization of muscle stem cells in post mortem tissue. (a) Enumeration by flow cytometry based on GFP expression of the number of viable satellite cells in one TA muscle fromTg:Pax7-nGFPmice (control, 2720±270 satellite cells; 1980±210 cells at 4, and 1040±230 at 8 days post mortem;n=5 mice, each time point). (b) Evaluation of viable cells in post mortem tissue by calcein incorporation (marker for all viable cells;n=7 mice), and satellite cells fromTg:Pax7-nGFPmice based on GFP expression (n=5 mice). (c) Enrichment of Pax7-expressing cells between day 0 and 4 post mortem indicated as percentage of X-gal+ cells fromPax7nlacZ/+animals, stained immediately in culture after isolation (n=10 mice). (d) Comparison of loss of satellite cells (Pax7-nGFP+ cells—black line) versus CD34+/Pax7-nGFP-/CD45- cells (containing fibroblasts, endothelial cells and non-satellite stem cells—grey line) (271,000±500 GFP+ cells versus 853,000±158,000 CD34+ cells at day 0 and 92,000±15,000 GFP+ cells versus 237,000±43,000 CD34+ cells 4 days post mortem) (n=3 mice). (e,f) Vimentin-positive fibroblasts cultured from CD34+/Pax7-nGFP-/CD45- cell fraction after sorting (n=3 mice per condition) (e) day 0 post mortem (f) 4 days post mortem; Bar, 50 μm. (g) Percentage of clonogenicity (number of cells forming colonies) after FACS and plating in 96-well dishes at day 0, 4 and 8 post mortem (n=5 mice per condition). (h) Evaluation by videomicroscopy (3% O2, 5% CO2) of time required to perform the first mitosis in cells from day 0, and 4 and 8 days post mortem (n=3 mice per condition). (i) Survival of quiescent or proliferating satellite cells post mortem. Satellite cells were enumerated by FACS from TA muscles of animals exposed to LPS (control, 6,100±1,700 satellite cells; 310±90 cells at 4 days post mortem;n=5 mice, each time point), or fromMdx4cv::Tg:Pax7-nGFPmice (7 months old) (control, 19,900±3,300 satellite cells; 2,400±390 cells at 4 days post mortem;n=9 mice, each time point), or following acute injury (5 days post-notexin injury) ofTg:Pax7-nGFPmice at day 0 or 4 days post mortem (pm) (control 5 days post-notexin, 103,000±8,500 satellite cells; 460±80 cells at 4 days post mortem;n=5 mice, each time point). Graphs indicate the percentage of viable satellite cells between day 0 and 4 days post mortem in the different cohorts. Statistical analysis was performed using paired or unpaired Student'st-tests, a minimum of 95% confidence interval for significance;P-values indicated on figures are <0.01 (**) and <0.001 (***). Figures display average values of all tests ± s.e.m. 1g and inset; 41–77 y.o., n =15; Table 2 ). Up to day 30 post sampling, the majority of the cultures (>80%) were myogenic as assessed by Myogenin + /Desmin + myotubes ( Fig. 1h,i ). After 30 days post sampling, viable cells were not obtained (assayed for 15 days in culture). Table 1 Biopsies from human cadavers. Full size table Figure 1: Skeletal muscle stem cells survive for extended periods post mortem. Tissue and cells from freshly sampled human biopsy ( a – c ). ( a ) Histology. Insets: immunostaining with satellite cell marker (CD56, brown). ( b ) Myotubes in vitro after 14 days culture from muscle biopsy (from same patient) expressing myogenin and desmin ( c ). Human deltoid muscle collected 17 days post mortem ( d – f ), ( d ) histology— inset is a CD56+ satellite cell, ( e ) myotube formation expressing myogenic markers ( f ). Muscle biopsy stored for 25 days post sampling (ps) from patient ( g – i ), ( g ) histology with a CD56+ satellite cell (inset), ( h ) myotube formation expressing myogenic markers ( i ). Mouse skeletal TA muscle 8 days post mortem ( j – l ) ( n =10 mice per time point). ( j ) Histology—inset satellite cell expressing M-Cadherin, ( k ) myotube formation, expressing myogenin and desmin ( l ). Note necrosis of haematoxylin and eosin (H&E)-stained myofibres ( d – j ). Histology figures are H&E stainings. Myotubes are stained with May Grünwald Giemsa (MGG) and immunostained with anti-myogenin (green), anti-desmin (red), and nuclei are counterstained with Hoechst (blue). Bar: 10 μm. Full size image Table 2 Biopsies from organ donors. Full size table Similar results were obtained with muscle stem cells (M-Cadherin-positive; Fig. 1j and inset) from mouse cadavers stored for 0–16 days at 4 °C. In all cases up to 10 days post mortem, myoblasts and differentiated cells were generated ( Fig. 1k, l ; n =10 mice per time point) as was the case for freshly isolated muscle stem cells. After this period, only some cultures yielded viable cells and myoblasts (80% of animals at day 12; 30% of animals at day 14; none at day 16; n =10 mice per time point), as microbial contamination during tissue decomposition increased considerably by later times thereby precluding further analysis. Muscle stem cells are enriched in post mortem tissue The number of muscle stem cells remaining in skeletal muscle post mortem was then enumerated by fluorescence-activated cell sorting (FACS) using Tg:Pax7-nGFP mice [10] . The paired/homeodomain transcription factor Pax7 is a marker of all satellite cells, and its expression is downregulated as myoblasts differentiate [9] , [11] , [12] , [13] . We compared the percentage of remaining satellite cells obtained from one Tibialis anterior (TA) muscle immediately after sacrifice and at different time points post mortem. Surprisingly, the percentage of satellite cells at 4 and 8 days post mortem was high (76.4±4.8% and 39.9±4%, respectively). Although this was reduced significantly by 12 and 16 days post mortem, satellite cells were reproducibly detected at these late time points (2.7±0.8% and 1.2±0.1% respectively; Fig. 2a ). All GFP + cells isolated by FACS were viable. To assess the relative ability of muscle stem cells to survive compared with other cell types, muscle cell suspensions were stained with calcein, which labels all living cells and enumeration was done by flow cytometry. At 4 days post mortem, 43% of the number of total cells were viable compared with 76% of satellite cells ( P <0.01; n =7 mice; Fig. 2b ). At 8 days post mortem, 10% of the number of total cells were viable compared with 40% of satellite cells ( P <0.001; n =7 mice; Fig. 2b ). Accordingly, a Pax7 nlacZ/+ knock-in mouse, which marks all satellite cells [14] , showed that between day 0 and 4 post mortem, the proportion of X-gal positive cells compared with all other cell types increased by 1.7-fold (31% at D0 and 53% at D4, P <0.001; n =10 mice per condition; Fig. 2c ). To assess whether other stem cells might also survive in post mortem muscle, CD45 − /CD34 + /GFP − cells, which contain interstitial multipotent mesenchymal stem cells as well as fibroblasts and endothelial cells [15] , [16] were isolated by FACS from Tg:Pax7-nGFP animals. The proportion of non-myogenic CD34 + cells decreased more dramatically than satellite cells between day 0 and day 4 post mortem (~82% decrease of CD45 − /CD34 + /GFP − cells; ~66% decrease of satellite cells; Fig. 2d ). Furthermore, culture of isolated CD45 − /CD34 + /GFP − cells failed to yield viable colonies with the exception of senescent fibroblasts ( Fig. 2e,f ). These findings are in keeping with recent reports demonstrating that other endogenous cell types fail to regenerate muscle after genetic ablation of satellite cells, thereby pointing to satellite cells as the central player in adult muscle regeneration [14] , [17] , [18] . Taken together, these findings provide evidence that muscle stem cells are preferentially enriched in post mortem tissue compared with other cell types. Figure 2: Characterization of muscle stem cells in post mortem tissue. ( a ) Enumeration by flow cytometry based on GFP expression of the number of viable satellite cells in one TA muscle from Tg:Pax7-nGFP mice (control, 2720±270 satellite cells; 1980±210 cells at 4, and 1040±230 at 8 days post mortem; n =5 mice, each time point). ( b ) Evaluation of viable cells in post mortem tissue by calcein incorporation (marker for all viable cells; n =7 mice), and satellite cells from Tg:Pax7-nGFP mice based on GFP expression ( n =5 mice). ( c ) Enrichment of Pax7-expressing cells between day 0 and 4 post mortem indicated as percentage of X-gal+ cells from Pax7 nlacZ/+ animals, stained immediately in culture after isolation ( n =10 mice). ( d ) Comparison of loss of satellite cells (Pax7-nGFP+ cells—black line) versus CD34+/Pax7-nGFP-/CD45- cells (containing fibroblasts, endothelial cells and non-satellite stem cells—grey line) (271,000±500 GFP+ cells versus 853,000±158,000 CD34+ cells at day 0 and 92,000±15,000 GFP+ cells versus 237,000±43,000 CD34+ cells 4 days post mortem) ( n =3 mice). ( e , f ) Vimentin-positive fibroblasts cultured from CD34+/Pax7-nGFP-/CD45- cell fraction after sorting ( n =3 mice per condition) ( e ) day 0 post mortem ( f ) 4 days post mortem; Bar, 50 μm. ( g ) Percentage of clonogenicity (number of cells forming colonies) after FACS and plating in 96-well dishes at day 0, 4 and 8 post mortem ( n =5 mice per condition). ( h ) Evaluation by videomicroscopy (3% O 2 , 5% CO 2 ) of time required to perform the first mitosis in cells from day 0, and 4 and 8 days post mortem ( n =3 mice per condition). ( i ) Survival of quiescent or proliferating satellite cells post mortem. Satellite cells were enumerated by FACS from TA muscles of animals exposed to LPS (control, 6,100±1,700 satellite cells; 310±90 cells at 4 days post mortem; n =5 mice, each time point), or from Mdx4cv::Tg:Pax7-nGFP mice (7 months old) (control, 19,900±3,300 satellite cells; 2,400±390 cells at 4 days post mortem; n =9 mice, each time point), or following acute injury (5 days post-notexin injury) of Tg:Pax7-nGFP mice at day 0 or 4 days post mortem (pm) (control 5 days post-notexin, 103,000±8,500 satellite cells; 460±80 cells at 4 days post mortem; n =5 mice, each time point). Graphs indicate the percentage of viable satellite cells between day 0 and 4 days post mortem in the different cohorts. Statistical analysis was performed using paired or unpaired Student's t -tests, a minimum of 95% confidence interval for significance; P -values indicated on figures are <0.01 (**) and <0.001 (***). Figures display average values of all tests ± s.e.m. Full size image Quiescence confers viability to post mortem stem cells Clonal analysis of muscle stem cells showed no significant difference in their ability to generate progeny between day 0 and day 4 post mortem samples (23.1% versus 16.3% clonogenicity, respectively). However, this value dropped markedly at day 8 (1.6%; Fig. 2g ). All colonies were myogenic as assessed by myotube formation and videomicroscopy ( Supplementary Movies 1–3 ). Notably, the exit from cell quiescence to perform the first cell division was significantly delayed in cells isolated from post mortem (29 h) compared with freshly sacrificed animals (21 h; Supplementary Movies 4, 5 ; Fig. 2h ), suggesting that the former are in a deeper state of quiescence. In spite of this delay, however, after the first division, myogenic cells divided every 7 h in low oxygen and synchronously in both conditions without any observable phenotypic differences indicating that this lag observed with post mortem animals is reversible. We then reasoned that the quiescent state might confer a survival advantage to the stem cells. To examine this possibility, four cohorts of mice were formed, where mice were treated as indicated or untreated, and then examined 4 days post mortem. In the first, the percentage of remaining satellite cells from uninjured TA muscle of Tg:Pax7-nGFP mice between 0 and 4 days post mortem was 76.4±4.8% ( n =5 mice, see Fig. 2a ). In the second cohort, mice were injected with bacterial lipopolysaccharide (LPS) to induce severe acute systemic inflammation. At 18 h after LPS injection, the percentage of viable satellite cells dropped dramatically to 5.1±2.3% ( n =5 mice, Fig. 2e ). In the third cohort, we used a mouse model of Duchenne muscular dystrophy, Mdx4cv , where chronic muscle degeneration and regeneration results in the continuous activation of satellite cells [19] , and crossed them with Tg:Pax7-nGFP mice. In this myopathy model, the TA muscle contained more myogenic cells than in normal mice during homoeostasis (20,000±3,200 versus 2,720±270 in control), reflecting the chronic regeneration and satellite cell mobilization. However, in spite of the higher initial numbers of myogenic cells in Mdx4cv mice, the percentage of remaining satellite cells between day 0 and day 4 post mortem in these animals was 14±3% ( n =9 mice, Fig. 2i ). In the fourth cohort, satellite cells were enumerated 5 days after a severe muscle injury with a myotoxin, thereby promoting stem cell re-entry into the cell cycle to effect myofibre regeneration [9] . At this time, myogenic cells proliferate actively (mean 103,000±8,500 GFP + /TA; n =5 mice, Fig. 2i ). In this cohort at 5 days post injury, mice were sacrificed, then satellite cells were enumerated by FACS at 4 days post mortem. The majority of these myogenic cells did not survive (0.45±0.1% remaining cells, n =5 mice; Fig. 2i ). Taken together, these experiments suggest that cellular quiescence, in part, protects stem cells from death in post mortem tissue. Downregulation of commitment markers in post mortem stem cells To assess the extent of lineage priming [20] and hence, the commitment status of the muscle stem cells post mortem, we performed RT–qPCR on satellite cells isolated by FACS. Cell determination and differentiation markers Myod and Myogenin , and the myofibre structural protein Troponin T were used as readouts for myogenic cell commitment, whereas Pax7 and the receptor stem cell marker CD34 were used as readouts of the more stem-like state [11] , [21] , [22] , [23] . Interestingly, a progressive increase in the levels of CD34 was observed from day 0 to day 8 post mortem, whereas an inverse trend was noted for Myod , Myogenin and Troponin T transcript levels ( n =5 mice; Fig. 3a ). This suggests that post mortem-derived muscle stem cells are less transcriptionally primed for myogenic commitment, thus they adopt a more stem-like state. To examine these cells in more detail, RT–qPCR analysis was performed on a number of genes involved in oxidative stress, hypoxia and apoptosis. Notably, the potent antioxidant glutathione peroxidase 1 [24] , the cell cycle exit regulator p21 [25] , the transcription factor and regulator of cell survival on oxidative stress, Foxo1 [26] , hypoxia-inducible factor 3a2 [27] , a transcription factor that regulates the adaptive responses to hypoxia, and angiopoietin 1, which promotes muscle stem cell quiescence [28] , were all upregulated in expression in post mortem muscle stem cells. In addition, the tumour suppressor p53 , which upregulates p21 , and is involved in a variety of stress responses [29] , was significantly upregulated in post mortem muscle stem cells, as was Ptx3 [30] , which is part of the inflammatory response and has a role at the late phase of apoptosis. However, no significant changes in expression of pro- and anti-apoptotic genes, such as Bax and Bcl2 , and other members of these families were noted ( Fig. 3b ). The transcription factor family NF-κB is a major regulator of cellular stress in a variety of contexts [31] , [32] . Expression of nfκb1 encoding NF-κB precursor of p50, p105, which is itself an NF-κB target gene, was significantly reduced in post mortem satellite cells compared with normal satellite cells, whereas levels of NF-κB p65 were unchanged ( Fig. 3b ). No translocation of p65 in the nucleus, indicative of NF-κB activation, was detected in normal and post mortem satellite cells, whereas normal satellite cells were able to activate NF-κB after stimulation with LPS, IL1β, TNF-α or during the isolation procedure itself (data not shown). To confirm these observations, two independent NF-κB-lacZ reporter transgenic mice were used [33] . NF-κB activity revealed by the presence of nuclear β-galactosidase was restricted to endothelial cells and a few interstitial cells with a fibroblast or smooth muscle cell phenotype ( Fig. 3c,d ). After 4 and 8 days post mortem, the number of β-galactosidase-positive cells decreased dramatically due to extensive cell death in the tissue. Notably, no detectable β-galactosidase-positive staining was observed in satellite cells ( Fig. 3e–h ). 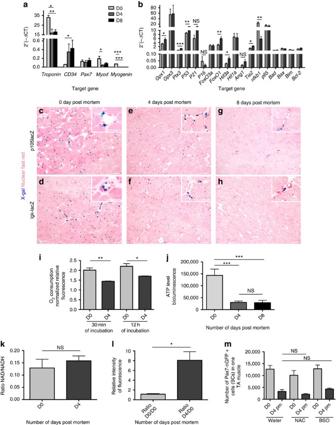Figure 3: Molecular characterization of viable muscle stem cells and redox status. (a,b) Real-time quantitative PCR of satellite cells (n=5 animals). (c–h) NF-κB activity in post mortem and anoxic satellite cells (in all experimentsn=5 mice). (c,d) Histology of normal muscle showing lacZ expression only in endothelial cells and some fibroblastic interstitial cells (blue nuclei) (haematoxylin and eosin (H&E) staining) using both p105lacZ transgenic mice (c) and Igkappa-lacZ (d). (e,f) 4 days post mortem, (g,h) 8 days post mortem, note reduction in lacZ-expressing cells, and no expression in cells in satellite cell position adjacent to myofibres. (i) Comparison of oxygen consumption between cells extracted 0 or 4 days post mortem after 30 min or 12 h in culture (n=5 mice). (j) Level of ATP in day 0, 4 and 8 post mortem satellite cells determined by fluorescence using luciferase activity (n=5 mice). (k) Determination of the ability to transform energy and the redox state ratio between NAD and NADH in cells freshly isolated or extracted 4 days post mortem (n=5 mice). (l) Measurement of the level of ROS in satellite cells expressed as a ratio between day 0 and 4 days post mortem (n=5 mice). (m) Enumeration of satellite cells at 0 and 4 days post mortem after variation of antioxidants in the satellite cell environment, by treatingTg:Pax7-nGFPmice withN-acetyl-L-cysteine (NAC) or buthionine sulfoximine (BSO) (n=5 mice). Statistical analysis was performed using paired or unpaired Student'st-tests, a minimum of 95% confidence interval for significance;P-values indicated on figures are <0.05 (*), <0.01 (**), and <0.001 (***). Figures display average values of all tests ±s.e.m. Figure 3: Molecular characterization of viable muscle stem cells and redox status. ( a , b ) Real-time quantitative PCR of satellite cells ( n =5 animals). ( c – h ) NF-κB activity in post mortem and anoxic satellite cells (in all experiments n =5 mice). ( c , d ) Histology of normal muscle showing lacZ expression only in endothelial cells and some fibroblastic interstitial cells (blue nuclei) (haematoxylin and eosin (H&E) staining) using both p105lacZ transgenic mice ( c ) and Igkappa-lacZ ( d ). ( e , f ) 4 days post mortem, ( g , h ) 8 days post mortem, note reduction in lacZ-expressing cells, and no expression in cells in satellite cell position adjacent to myofibres. ( i ) Comparison of oxygen consumption between cells extracted 0 or 4 days post mortem after 30 min or 12 h in culture ( n =5 mice). ( j ) Level of ATP in day 0, 4 and 8 post mortem satellite cells determined by fluorescence using luciferase activity ( n =5 mice). ( k ) Determination of the ability to transform energy and the redox state ratio between NAD and NADH in cells freshly isolated or extracted 4 days post mortem ( n =5 mice). ( l ) Measurement of the level of ROS in satellite cells expressed as a ratio between day 0 and 4 days post mortem ( n =5 mice). ( m ) Enumeration of satellite cells at 0 and 4 days post mortem after variation of antioxidants in the satellite cell environment, by treating Tg:Pax7-nGFP mice with N -acetyl- L -cysteine (NAC) or buthionine sulfoximine (BSO) ( n =5 mice). Statistical analysis was performed using paired or unpaired Student's t -tests, a minimum of 95% confidence interval for significance; P -values indicated on figures are <0.05 (*), <0.01 (**), and <0.001 (***). Figures display average values of all tests ±s.e.m. Full size image Lower metabolism and higher ROS in post mortem stem cells To investigate further the mechanisms associated with muscle stem cell survival, we compared oxygen consumption between satellite cells extracted 0 and 4 days post mortem. Interestingly, oxygen consumption was 28% lower after 30 min in culture in 4 days post mortem-extracted cells compared with those isolated at D0, and this value remained reduced (23%) after 12 h in culture ( Fig. 3i ). Accordingly, the level of ATP was significantly diminished in post mortem stem cells compared with those at D0, and these values were not altered significantly between day 4 and 8 post mortem ( Fig. 3j ). NAD + and NADH are mediators of the cellular energy metabolism and the cellular NAD + /NADH ratio is an index of the reduction–oxidation (redox) equilibrium that reflects both the metabolic activities and the health of cells [34] . A measure of the NAD + /NADH ratio in satellite cells showed no significant difference between 0 and 4 days post mortem indicating no change in the redox state of post mortem stem cells ( Fig. 3k ). Interestingly, the level of ROS was elevated 8-fold in satellite cells extracted 4 days post mortem compared with freshly isolated cells ( Fig. 3l ). To extend this observation, three cohorts of Tg:Pax7-nGFP mice received water or a daily administration of the glutathione donor N -acetyl- L -cysteine for 1 week to protect against ROS, or buthionine sulfoximine for 15 days to deplete glutathione within cells as previously described [35] , [36] . The number of satellite cells that survived 4 days post mortem was not significantly different within these three sets of mice ( Fig. 3m ). Taken together, these results indicate that surviving satellite cells are in a low metabolic state, consume less oxygen, and produce lower levels of ATP. In addition, in spite of higher levels of ROS in post mortem muscle stem cells, the cellular redox state remained stable. To extend these observations, we modelled elements of the hostile post mortem environment by examining anoxia in low temperature. Post mortem muscle stem cells isolated from Tg:Pax7-nGFP mice were incubated for up to 21 days at 4 °C in anoxic GenBag chambers (less than 0.1% oxygen). Strikingly, muscle stem cells survived significantly better in this anoxic environment compared with cells incubated in atmospheric oxygen (21%) at 4 °C ( Fig. 4a ). After 4 days at 4 °C, ~82% of satellite cells were lost in normoxia compared with ~29 % in anoxia ( P <0.01; n =7 mice; Fig. 4a ). These muscle stem cells retained their capacity to differentiate after several days without oxygen ( Fig. 4b,c ). In marked contrast to post–mortem-derived satellite cells, cells maintained in anoxic conditions had ~9-fold reduced levels of ROS compared with normal cells ( Fig. 4d ). 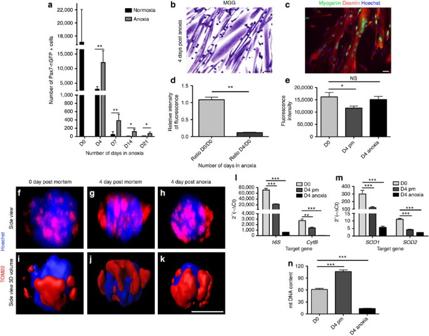Figure 4:In vitromodelling of anoxia and mitochondrial status of muscle stem cells. (a) Satellite cells were isolated by FACS from day 0, cultured at 4°C in normoxia or anoxia, then enumerated at indicated times (n=7 mice); (b,c)in vitroassessment of myotube formation and expression of myogenic markers Myogenin and Desmin with satellite cells cultured in anoxia (n=5 mice). (d) Measurement of ROS of cells that remain alive after 4 days in anoxia. Ratio between day 0, and 4 days in anoxia; (n=5 mice). (e) Fluorescence intensity quantification of TOM22 immunolabelling per cell in freshly isolated cells, in cells extracted 4 days post mortem and 4 days in anoxia (n=30 cells;n=4 mice per condition). (f–k) 3D imaging of mitochondrial mass in satellite cells (n=4 mice). (f,i) day 0; (g,j) 4 days post mortem; (h,k) 4 days post anoxia. Immunolabelling shown for mitochondria with TOM22 (red), and nuclei (blue) with Hoechst 33342. For each condition, side view and 3D volume rendering are shown; 360° view of these cells is shown inSupplementary Movies 6–8. (l) RT–qPCR of mitochondrial genes,16SrRNA andCytB(n=6 mice). mt rRNA is present in greater amounts than mRNA, as expected58,59. (m) RT–qPCR of SOD1 and SOD2 (n=6 mice). (n) mtDNA content (12Sregion) estimation by qPCR (n=6 mice). Statistical analysis was performed using paired or unpaired Student'st-tests, a minimum of 95% confidence interval for significance;P-values indicated on figures are <0.05 (*), <0.01 (**), and <0.001 (***). Figures display average values of all tests ±s.e.m. Figure 4: In vitro modelling of anoxia and mitochondrial status of muscle stem cells. ( a ) Satellite cells were isolated by FACS from day 0, cultured at 4°C in normoxia or anoxia, then enumerated at indicated times ( n =7 mice); ( b , c ) in vitro assessment of myotube formation and expression of myogenic markers Myogenin and Desmin with satellite cells cultured in anoxia ( n =5 mice). ( d ) Measurement of ROS of cells that remain alive after 4 days in anoxia. Ratio between day 0, and 4 days in anoxia; ( n =5 mice). ( e ) Fluorescence intensity quantification of TOM22 immunolabelling per cell in freshly isolated cells, in cells extracted 4 days post mortem and 4 days in anoxia ( n =30 cells; n =4 mice per condition). ( f – k ) 3D imaging of mitochondrial mass in satellite cells ( n =4 mice). ( f , i ) day 0; ( g , j ) 4 days post mortem; ( h , k ) 4 days post anoxia. Immunolabelling shown for mitochondria with TOM22 (red), and nuclei (blue) with Hoechst 33342. For each condition, side view and 3D volume rendering are shown; 360° view of these cells is shown in Supplementary Movies 6–8 . ( l ) RT–qPCR of mitochondrial genes, 16S rRNA and CytB ( n =6 mice). mt rRNA is present in greater amounts than mRNA, as expected [58] , [59] . ( m ) RT–qPCR of SOD1 and SOD2 ( n =6 mice). ( n ) mtDNA content ( 12S region) estimation by qPCR ( n =6 mice). Statistical analysis was performed using paired or unpaired Student's t -tests, a minimum of 95% confidence interval for significance; P -values indicated on figures are <0.05 (*), <0.01 (**), and <0.001 (***). Figures display average values of all tests ±s.e.m. Full size image Given our findings above regarding the metabolic and oxidative state of satellite cells, we examined in detail the mitochondrial status of satellite cells in post mortem and anoxic scenarios. Here, 0 and 4 days post mortem satellite cells were immunolabelled to detect TOM22, a core component of the mitochondrial outer membrane translocase [37] , as a readout of mitochondrial mass. We observed a decrease of 28.3% in mitochondrial mass in 4 days post mortem but not in 4 days anoxia-treated cells compared with freshly isolated cells ( n =30 cells from four mice, Fig. 4e ). With 3D analysis, the overall organization of the mitochondrial network seemed comparable under these conditions ( Fig. 4f–k , Supplementary Movies 6–8 ). Moreover, RT–qPCR analysis of mitochondrial mRNA ( CytB ) and rRNA ( 16S ) revealed significantly decreased steady-state levels of these transcripts in 4 days post mortem and, to a greater extent, in 4 days anoxia-treated satellite cells, compared with the control ( Fig. 4l ). We also observed decreased expression of the nuclear encoded CuZn-SOD1 and Mn-SOD2 super oxide dismutases, which are important components of the cellular antioxydant defence mechanism, in 4 days post mortem and in 4 days anoxia-treated cells compared with control cells ( Fig. 4m ). These findings are in agreement with previous reports noting a decline in mitochondrial RNAs and antioxidant SOD enzymes in a low-oxygen environment [38] , [39] . Interestingly, we noted a significant increase by 57.8% of the mitochondrial DNA (mtDNA) content in 4 days post mortem muscle stem cells. In contrast, mtDNA content decreased dramatically (78.1%) in 4 days anoxia-treated cells ( Fig. 4n ). Taken together, these findings indicate that although anoxia mimics under certain conditions the post mortem scenario, differences in oxygen consumption, ROS activity and mtDNA content suggest that stem cell behaviour under these conditions are not identical, and that perhaps residual levels of oxygen are present in post mortem tissue. Engraftment potential of post mortem mouse muscle stem cells To evaluate the regenerative potential of muscle stem cells after transplantation, and consequently the reversibility of the dormant cell state in vivo , satellite cells were isolated by FACS from triple transgenic donor mice, Tg:Pax7-nGFP::Tg:CAG-PLAP::Tg:MLC3F-nlacZ-2E . The ubiquitous PLAP (human placental alkaline phosphatase) reporter marks all transplanted cells, whereas nlacZ expression from the myosin light chain promoter marks differentiated cells [10] . GFP + cells were isolated from 0 or 4 days post mortem skeletal muscles, or cells were maintained at 4 °C without oxygen for 4 days, then transplanted into cardiotoxin pre-injured regenerating TA skeletal muscles of immunocompromised Rag2 −/− :γ C −/− recipient mice [10] ( n =5 recipient mice total; Fig. 5a–d ). Transplantation of 5,000 satellite cells from day 4 post mortem donor mice or satellite cells maintained for 4 days in anoxia yielded and average of 75 and 69 PLAP-expressing myofibres/TA muscle, respectively, with centrally located nuclei (a hallmark of regeneration) [9] ( Fig. 5b–d ). Notably, the number of regenerating fibres was equivalent, or slightly higher that those obtained with control freshly isolated satellite cells (54 PLAP expressing-myofibres; Fig. 5a,d ). Given that efficient regeneration by satellite cells is directly influenced by endothelial cells and the extent of vessel formation [8] , we enumerated the number of capillary sections around each donor-derived myofiber to examine the extent of vessel formation. No significant differences were observed among regenerated myofibers indicating that the ability to stimulate capillaries was not hampered by post mortem or anoxic-derived satellite cells ( Fig. 5e ). 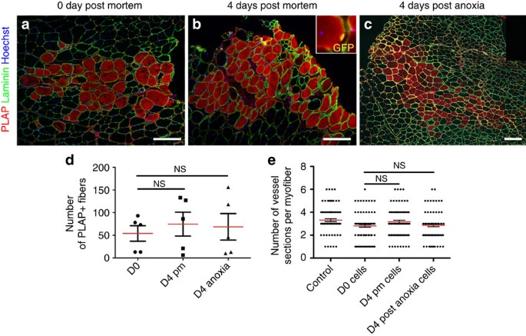Figure 5: Muscle stem cells that survive post mortem or in anoxia retain robust regenerative potential after transplantation. (a–c) Transplantation of muscle stem cells fromTg:Pax7-nGFP::Tg:CAG-PLAP::Tg:MLC3F-nlacZ-2Edonor mice into pre-injured TA muscle of immunocompromised recipient mice (n=5 mice). Immunohistochemistry showing contribution of donor-transplanted stem cells to regenerating fibres (red) in recipient mouse; inset inbshows a satellite cell in the niche after self-renewal. (d) Number of myofibres engrafted in the recipient muscle after injection of 5000 freshly isolated, post mortem, or anoxic donor cells (n=5 recipient mice each; 54±17 PLAP positive fibres with freshly isolated cells, 75±26 with 4 days post mortem cells, 69±29 with anoxic donor cells). (e) Distribution of the number of capillary sections around myofibers after regeneration in non-engrafted regenerated fibers (centrally nucleated), engrafted (hPLAP-positive) with 4 days post mortem or 4 days post anoxia donors. Statistical analysis was performed using paired or unpaired Student'st- tests, a minimum of 95% confidence interval for significance. Figures display average values of all tests ±s.e.m. Figure 5: Muscle stem cells that survive post mortem or in anoxia retain robust regenerative potential after transplantation. ( a – c ) Transplantation of muscle stem cells from Tg:Pax7-nGFP::Tg:CAG-PLAP::Tg:MLC3F-nlacZ-2E donor mice into pre-injured TA muscle of immunocompromised recipient mice ( n =5 mice). Immunohistochemistry showing contribution of donor-transplanted stem cells to regenerating fibres (red) in recipient mouse; inset in b shows a satellite cell in the niche after self-renewal. ( d ) Number of myofibres engrafted in the recipient muscle after injection of 5000 freshly isolated, post mortem, or anoxic donor cells ( n =5 recipient mice each; 54±17 PLAP positive fibres with freshly isolated cells, 75±26 with 4 days post mortem cells, 69±29 with anoxic donor cells). ( e ) Distribution of the number of capillary sections around myofibers after regeneration in non-engrafted regenerated fibers (centrally nucleated), engrafted (hPLAP-positive) with 4 days post mortem or 4 days post anoxia donors. Statistical analysis was performed using paired or unpaired Student's t - tests, a minimum of 95% confidence interval for significance. Figures display average values of all tests ±s.e.m. Full size image Engraftment of post mortem mouse HSCs To investigate whether our findings can be extended to another stem cell model, blood stem and progenitor cells were examined. At 2 and 4 days post mortem, bone marrow (BM) was severely altered showing cell compaction, shrinkage of cytoplasm and oedema ( Fig. 6a–c ). At daily intervals post mortem, the BM of Tg:CAG-GFP mouse femur was flushed and the engraftment potential of transplanted progenitors was assessed. Survival of BM cells after storage in anoxia was determined ( Fig. 6d ). Full reconstitution was observed in lethally irradiated C57BL/6 recipient mice ( n >5 mice per time point; Fig. 6e black bars). GFP+ leukocytes were found in all lineages (B and T lymphocytes, granulocytes or monocytes using B220 and CD5, Gr1 Ly6C or CD11b expression, respectively) as assessed by flow cytometry ( Fig. 6f ). To determine if post mortem BM contained long-term HSCs, serial transplantations were performed with the grafted BM in lethally irradiated recipient mice. In all cases (day 2, 3 or 4 days post mortem), all of the animals were viable with 100% chimerism ( Fig. 6e , grey bars). Similar results were obtained with HSCs kept in anoxia. BM cells were extracted from Tg:CAG-GFP mice and kept at 4 °C for 1–4 days in anoxia, and transplanted into lethally irradiated C57BL/6 recipient mice ( n ≥5 mice per condition). Whereas, the number of cells remaining was low (36.5±5.6 at day 1 and 4.4±0.8 at day 4 post anoxia, Fig. 6d ), mice survived after BM transplantation, chimerism was 100% ( Fig. 6g , black bars) and all haematopoietic lineages were reconstituted ( Fig. 6h ). Serial transplantations of BM cells isolated after the first round of transplantation demonstrated that the HSCs can repopulate all lineages in the blood ( Fig. 6g , grey bars). 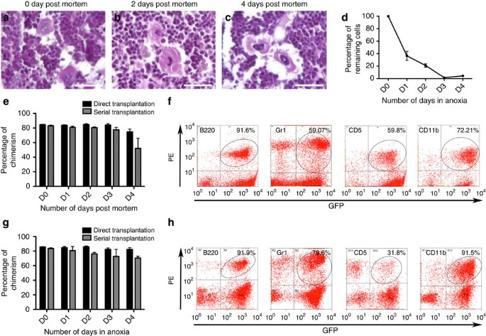Figure 6: HSC that survive post mortem or in anoxia retain robust regenerative potential after transplantation. (a) Histology of normal mouse BM (H&E staining;n=5 mice). (b,c) Histology of mouse cadaver BM (2 and 4 days post mortem) showing cell compaction, shrinkage of cytoplasm and oedema (H&E staining after decalcification and paraffin embedding). (d) Percentage of viable whole BM cells several days after storage at 4 °C in anoxia (cell viability assessed by trypan blue exclusion;n=5 mice). (e) Blood chimerism (% of GFP+ cells in circulating blood) in mice post-irradiation and BM transplantation with BM extracted from one femur and collected 0, 1, 2, 3 and 4 days post mortem (n>5 mice per condition). Black bars indicate results with a single BMT, grey bars after one serial transplantation. (f) Immunophenotyping of circulating GFP+ cells after serial BMT showing GFP+ B cells (B220 staining), GFP+ T cells (CD5 staining), GFP+ granulocytes (Gr1 staining), and GFP+ monocytes (CD11b Staining). (g) Reconstitution with BM maintained several days in anoxia. Blood chimerism (% of GFP+ cells in circulating blood) in surviving mice post irradiation and BMT with BM cells kept at 4 °C and in anoxia for 0, 1, 2, 3, 4 days (n> 5 mice per condition). Black bars indicate results with a single BMT and grey bars after one serial transplantation. (h) Reconstitution of all white blood cells lineages as assessed by presence of GFP+ B cells (B220 staining), GFP+ T cells (CD5 staining), GFP+ granulocytes (Gr1 staining) and GFP+ myeloid cells (CD11b staining). Figures display average values of all tests ±s.e.m. Figure 6: HSC that survive post mortem or in anoxia retain robust regenerative potential after transplantation. ( a ) Histology of normal mouse BM (H&E staining; n =5 mice). ( b , c ) Histology of mouse cadaver BM (2 and 4 days post mortem) showing cell compaction, shrinkage of cytoplasm and oedema (H&E staining after decalcification and paraffin embedding). ( d ) Percentage of viable whole BM cells several days after storage at 4 °C in anoxia (cell viability assessed by trypan blue exclusion; n =5 mice). ( e ) Blood chimerism (% of GFP+ cells in circulating blood) in mice post-irradiation and BM transplantation with BM extracted from one femur and collected 0, 1, 2, 3 and 4 days post mortem ( n >5 mice per condition). Black bars indicate results with a single BMT, grey bars after one serial transplantation. ( f ) Immunophenotyping of circulating GFP+ cells after serial BMT showing GFP+ B cells (B220 staining), GFP+ T cells (CD5 staining), GFP+ granulocytes (Gr1 staining), and GFP+ monocytes (CD11b Staining). ( g ) Reconstitution with BM maintained several days in anoxia. Blood chimerism (% of GFP+ cells in circulating blood) in surviving mice post irradiation and BMT with BM cells kept at 4 °C and in anoxia for 0, 1, 2, 3, 4 days ( n > 5 mice per condition). Black bars indicate results with a single BMT and grey bars after one serial transplantation. ( h ) Reconstitution of all white blood cells lineages as assessed by presence of GFP+ B cells (B220 staining), GFP+ T cells (CD5 staining), GFP+ granulocytes (Gr1 staining) and GFP+ myeloid cells (CD11b staining). Figures display average values of all tests ±s.e.m. Full size image We show that muscle stem cells have a remarkable ability to survive for extended periods post mortem, in both humans and mice. Significantly, post mortem skeletal muscle and HSCs maintain their functional properties in vitro and after transplantation, or after prolonged storage in anoxia. It is generally thought that stem cells lose their potential and utility for experimental and clinical purposes within 24–48 h post mortem in the necrotic environment of the cadaver, and several studies have reported that neural and HSCs can survive within this time interval [1] , [2] , [3] , [4] , [6] , [7] , [40] . Here we describe culture conditions that permit the survival of two stem cell types for remarkably longer periods post mortem than previously described, while retaining full engraftment potential. We propose that the lack of oxygen, nutrients, or the presence of extensive necrosis triggers a cellular response in stem cells resulting in their adopting a deeper state of quiescence or dormancy. A similar phenomenon was described in yeast where removal of essential nutrients induces quiescence [41] . Interestingly, it was reported that a subpopulation of HSCs that divide infrequently are in a dormant reversible cell state [42] . We also reported recently that a subpopulation of quiescent muscle stem cells corresponding to high Pax7-nGFP expression are in deeper quiescence, or dormant [23] . Whether these dormant cells are subsequently enriched in post mortem muscles awaits further experimentation. Satellite cells isolated from 4 days post mortem muscle display reduced mitochondrial mass, reduced transcription of mitochondrial and antioxidant genes and increased mtDNA content, compared with normal cells. These characteristics seem to be a consequence of decreased oxygen tension. Indeed, hypoxia leads to about 30% loss of mitochondrial density in skeletal muscle [43] , to an increase of mtDNA content [44] , and to generation of ROS [45] to which the reduced anti-oxidant activity might contribute. Interestingly, low-oxygen tension equivalent to hypoxia is prevalent in the muscle stem cell niches [46] as in other stem cell niches (for example, haematopoietic, mesenchymal and neural stem cells) [47] . The high levels of ROS that we report in post mortem stem cells might signal their susceptibility to death. However, recent evidence points to a role for ROS in cell fate determination in Drosophila [48] , and studies in C. elegans found that ROS is associated with cell survival [49] . Interestingly, we report also that the high levels of ROS in post mortem muscle stem cells was coincident with relatively unchanged redox levels. This was in striking contrast to the dramatically reduced levels of ROS noted in muscle stem cells stored in anoxia. Notably, whereas ROS are considered as potent activators of NF-κB [50] , we report that NF-κB is not activated, and even slightly reduced, in post mortem muscle stem cells. These findings suggest that in post mortem muscle stem cells ROS may have an inhibitory effect on NF-κB activation as described thus far only in lung epithelial cells [51] . Interestingly, distinct phenotypic outcomes including quiescence or proliferation, and apoptosis or survival, have been suggested to be modulated by severe or mild hypoxic conditions (0.1–1%) [52] , or the bioenergetic requirement of the cell [53] . Our findings suggest that this might also be the case as the degree of hypoxia/anoxia in dormant muscle stem cells could maintain their viability for unusually long periods in spite of the necrotic microenvironment. The reduction of mitochondrial and antioxidant gene transcription was exacerbated in day 4 –anoxia-treated cells that also display a dramatic reduction of the mtDNA content, without alterations of the mitochondrial mass. These characteristics are compatible with the shift from hypoxia to anoxia, where mitochondria switch from producers to consumers of ATP without changing their mitochondrial mass [54] . Moreover, the mtDNA content and mtRNA levels decrease when mitochondria cease their energy production [55] . Taken together, these data indicate that day 4-anoxia-treated satellite cells display the hallmarks of anoxic mitochondria, and suggest that day 4 post mortem satellite cells might not be in an truly anoxic microenvironment. It would be interesting to examine mild and severe hypoxic microenvironments in relation to stem cell viability in future studies. In the haematopietic system, quiescence is associated with the absence of productive mRNA transcription [56] but also maintenance of energy homoeostasis that restricts entry into the cell cycle [53] , [57] . The lowering of mitochondrial activity in post mortem muscle stem cells is directly associated with, and likely promotes the dormant cell state. Notably, this state of dormancy is reversible and normal cell cycle kinetics resume after revival, both in culture and after transplantation in vivo . The resistance to severe hypoxia, which we observe in cadavers and in vitro could be considered either as an intrinsic characteristic of a subpopulation of stem cells, or a general mechanism of all stem cells, which have developed the capacity to reduce their metabolic activity and adopt a more stem cell state under extreme conditions of stress. Ethical Human samples were collected according to guidelines recommended by the national ethical committee. All mice were housed in a level 2 biosafety animal facility. Before manipulations, animals were anaesthetized using intraperitoneal injection of Ketamine and Xylazine (respectively, 25% and 12.5%, in phosphate-buffered saline (PBS)). This study was conducted in accordance with the local and EC guidelines for animal care [Journal Officiel des Communautés Européennes, L358, december 18, 1986]. Mouse strains and treatments C57BL/6, Tg:CAG-GFP (ref. 60 ), Mdx4cv (ref. 9 ), p105-lacZ, Igkappa-lacZ (ref. 33 ) mice were used. Myoinjury was induced by injection of 10 μl notexin (12.5 μg ml −1 Latoxan, France) in TA muscles. Mice were treated via intraperitoneal injection of 100 μl with LPS (from Escherichia coli 055:B5; 75 mg kg −1 , Sigma) and sacrificed 19 h post treatment. Mice received L -buthionine (S,R)-sulfoximine (Sigma-Aldrich, Saint-Louis, MO, USA), an inhibitor of glutathione synthesis, in the drinking water as described previously [36] at a concentration of 5 mg ml −1 (average dose of 185 mg kg −1 per day) for 14 days to continuously [35] deplete levels of GSH. Mice received the glutathione precursor N -acetylcysteine (Sigma) in the drinking water (140 mg kg −1 per day) for 1 week. Bone marrow transplantation For BM transplantations, donor BM cells were obtained by flushing two femurs of donor mice (various times post mortem) with RPMI medium (Invitrogen, Paisley, UK) and 5 IU ml −1 heparin (Sanofi, France). In the case of late post mortem cadavers the BM cell suspension was incubated with 50 μg ml −1 DNAse I (Roche, Mannheim, Germany) to preclude clotting of cells. After washing, retro-orbital injection of cells was done in 0.1 ml fresh mouse serum and Hanks Buffer (PAA Laboratories GmbH, Pasching, Austria) (1:1), in 95 cGy-irradiated, 8-week-old C57BL/6 mice ( 60 Co γ rays within 1 day before BM transplantation). After transplantation, mice received 10 mg kg −1 per day ciprofloxacin for 10 days to prevent infection during the aplastic phase. Tissue specimens Cadavers were stored at 4 °C after a variable period lasting from several hours to 12 h at room temperature between death and transportation to a funerary room. Biopsies were obtained from organ donors at the time of disconnection of the patient from the respirator during the procedure of organ sampling. Histopathological examination of these biopsies did not show specific pathology. A biopsy (4 g) was isolated from the Deltoid or the Quadriceps muscle 6–17 days post mortem in cadavers or from psoas or intercostals in organ donors. All human and mouse tissues were frozen in isopentane cooled by liquid nitrogen before cryosectionning (5 μm). Immunohistochemistry The following primary antibodies were used: mouse monoclonal antibodies against human Placental Alkaline Phosphatase (8B6) (1:300, GenTex, Irvine, CA, USA), M-cadherin (1:50, Alexis Biochemicals, Lausen, Switzerland) and mouse monoclonal antibodies against human Myogenin (1:50, BD Pharmingen, San Jose, CA, USA), rabbit polyclonal antibodies against human Desmin (1:50, Abcam, Cambridge, UK), rat anti-mouse Myogenin (1:50, Santa Cruz biotechnologies, Santa Cruz, CA, USA) and mouse Laminin-2 (1:50, Sigma). Secondary antibodies were Cy3 donkey anti-mouse (1:400, Jackson Immunoresearch lab, Baltimore, PA, USA), FITC goat anti-mouse (1:200, Jackson), Cy3 donkey anti-rabbit (1:200, Jackson), biotinylated horse anti-mouse (1:200, Vector laboratories, Burlingame, CA, USA), Cy5 donkey anti-rabbit (1:200, Jackson) and DTAF-streptavidin (1:400, Immunotech Beckman, Brea, CA, USA). A classical protocol was used: rehydratation, blocking with 20% goat serum and 0.5% Triton-X 100 for 20 min, incubation with primary antibody (Dako Diluent buffer; Glostrup, Denmark) overnight at 4 °C, and incubation with secondary antibody incubated 1 h at 37°C. For X-gal staining, tissues or cells were incubated in a solution containing 4 mM each of potassium ferrocyanide, potassium ferricyanide, 2 mM MgCl 2 , 400 μg ml −1 X-gal, and 0.02% NP40 in PBS at 32 °C for various times. For evaluation of mitochondrial mass, 20,000 fixed cells in suspension were permeabilized (0.5% Triton X-100), incubated in blocking buffer (bovine serum albumin 5%; 1× PBS) for 1 h, incubated with primary rabbit anti-TOM22 antibody (HPA003037; Sigma) for 1 h, revealed with Alexa-555 anti-rabbit antibody (Invitrogen). All slides were counterstained with 10 μg ml −1 Hoechst 33342 (Sigma). Imaging Bright field and fluorescence microscopy were peformed using a Zeiss Axiophot microscope. Confocal acquisitions were performed using a spinning-disk Perkin-Elmer Ultraview RS Nipkow Disk (laser-scanning confocal microscope Zeiss Axiovert 200 M, 100×/1.4 objective and a Hamamatsu ORCA II ER camera). Optical slices were taken every 200-nm interval along the z -axis covering the whole depth of the cell, at resolution of 1.024/1.024 pixels. Image reconstructions were achieved using the IMARIS software (Bitplane) and image analysis using ImageJ 1.34-s software. Live videomicroscopy Cells were plated immediately after sorting in a 24-well Matrigel-coated plate with a glass bottom (MatTek) in a drop of pre-equilibrated medium (1:1 DMEM Glutamax: MCDB (Sigma), 20% FCS overnight. The next day, cells were filmed using a Zeiss inverted Axio Observer Z1 microscope with a LCI PlnN 10×/0.8 W DICII objective, a Colibri light source and an incubation chamber at 37 °C, 5% CO 2 , 3% O 2 . Live cells were monitored every 20 min with Bright field and DICII filters and Axiovision software. To increase the field, MozaiX was used (3X3) and both wells were imaged simultaneously using the Mark and Find module. Cell culture In standard conditions, cells were grown in Ham's F12 medium containing 20% FCS 1% UltroserG (PALL Life Sciences, France), 0.2% vitamins, 0.4% Penicillin Streptomycin 10,000 U ml −1 . In differentiating conditions, growth medium was replaced by Ham's F12 medium containing 5% FCS at time of subconfluence. Unless otherwise indicated, culture media components were obtained from Gibco (Invitrogen) and culture plastics were obtained from TPP (Trasadingen, Switzerland). To activate the NF-κB signalling pathway, cells were treated for 10 min, 30 min or 1 h either with mouse tumour necrosis factor-α at 10 ng ml −1 (R&D Systems), human interleukin-1β at 20 ng ml −1 (R&D Systems), lymphotoxin α/β at 1 μg ml −1 (Sigma) and for 1 h, 4 h or 24 h with LPS at 40 ng ml −1 (Sigma). Flow cytometry MoFlo Legacy (Beckman Coulter, Brea, CA, USA) was used for cell sorting and CyAn ADP for cell analysis (Beckman Coulter). All analyses and quantitations were performed using Summit v4.3 software from DakoCytomation. In all these experiments, cells were also labelled with 1 μM propidium iodide (Sigma) to exclude dead cells from analysis. For the assessment of cell viability, cells were stained by calcein AM (Invitrogen) for 5 min at room temperature. The fluorescent probe CellROX deep Red Reagent (Invitrogen) was used to monitor the intracellular generation of ROS. Cells were incubated 30 min with CellROX deep red at 37 °C and fluorescence intensity was measured by FACS. To quantify the extent of engraftment, peripheral blood mononuclear cells of transplanted mice were analysed 1 month post transplantation. Leukocytes were gated on, and GFP fluorescence was measured, under the fluorescein isothiocyanate channel. Specific fluorescence stainings were done using phycoerythrin (PE)-Cy5-conjugated anti-Ly-6C (Gr1), PE-conjugated anti-CD11b, PE-conjugated anti-CD5, PE-conjugated anti-B220 antibodies and their respective isotypes (all from eBioscience, San Diego, CA, USA). ATP levels For measuring the levels of ATP, cells were isolated by FACS directly in lysis buffer and maintained at 4°C. An ApoSENSOR kit from Biovision (New Mountain, CA, USA) was used to measure ATP levels where luciferin reacts with ATP and emits signal in proportion to ATP content; emitted light was measured using a luminometer (GLOMAX 20/20, Promega). For all three conditions, 20,000 cells (isolated by FACS and verified by direct counting) were used. The quantity of ATP was determined by fluorescence using luciferase activity as a readout. NAD + /NADH and oxygen consumption The NAD + /NADH ratio was measured from isolated cells by FACS using the Biovision NAD+/NADH kit (#K337-100, Biovision). Oxygen consumption was established by using the fluorescent Oxygen Biosensor Systems (BD biosciences, Bedford, MA, USA). Normalized relative fluorescence units were obtained by dividing the fluorescence values of cells with the value of blank wells. Molecular biology Total DNA was prepared using extraction buffer (0.2 mg ml −1 proteinase K, 0.2% SDS and 5 mM EDTA) and incubated at 50°C for 3 h. DNA was precipitated with 3 M sodium acetate (pH 5.2) and isopropanol for 20 min on ice before centrifugation at 12,000 rpm at 4 °C. Real-time PCR amplification was performed on 200 pg of total DNA using the StepOne Plus RealTime PCR system (Applied Biosystems, Carlsbad, CA, USA) and Power Sybr Green PCR Master mix (ABI). A fragment of mitochondrial COI gene, the established marker for mtDNA content in mouse cells, was amplified using the nuclear encoded NDUFV1 gene as endogenous reference [59] . The level of mtDNA was calculated using the ΔCT of average CT of mtDNA and nDNA (ΔCT=CT nDNA − CT mtDNA) as 2ΔCT. Total RNA was extracted from cells isolated by FACS directly in lysis buffer using the RNAeasy Micro purification Kit (Qiagen, Germantown, PA, USA). RNA was processed for random-primed reverse transcription using the SuperScript II reverse transcriptase protocol of Invitrogen. The complementary DNAs were then analysed by real-time PCR using Taqman universal Master Mix and an ABI Prism 7700 and a StepOnePlus (Applied Biosystems). TBP reference transcript levels were used for the normalization of each target within each sample (=CT). Custom primers were designed using Primer3Plus online software ( http://www.bioinformatics.nl/cgi-bin/primer3plus/primer3plus.cgi ) ( Supplementary Table S1 ). Statistics Statistical analysis was performed with GraphPad Prism software using paired or unpaired Student's t -tests, a minimum of 95% confidence interval for significance; P -values indicated on figures are <0.05 (*), <0.01(**), and <0.001 (***). Figures display average values of all tests ±s.e.m. How to cite this article: Latil, M. et al . Skeletal muscle stem cells adopt a dormant cell state post mortem and retain regenerative capacity. Nat. Commun. 3:903 doi: 10.1038/ncomms1890 (2012).